Pair distribution function computed tomography An emerging theme of modern composites and devices is the coupling of nanostructural properties of materials with their targeted arrangement at the microscale. Of the imaging techniques developed that provide insight into such designer materials and devices, those based on diffraction are particularly useful. However, to date, these have been heavily restrictive, providing information only on materials that exhibit high crystallographic ordering. Here we describe a method that uses a combination of X-ray atomic pair distribution function analysis and computed tomography to overcome this limitation. It allows the structure of nanocrystalline and amorphous materials to be identified, quantified and mapped. We demonstrate the method with a phantom object and subsequently apply it to resolving, in situ , the physicochemical states of a heterogeneous catalyst system. The method may have potential impact across a range of disciplines from materials science, biomaterials, geology, environmental science, palaeontology and cultural heritage to health. Complex heterogeneous systems of nanostructured materials are at the heart of next-generation technologies in sustainable energy, environmental remediation and health [1] . To understand how the materials perform under realistic conditions it is necessary to study them in situ , which in general means examining the evolution of nanostructures within complex mixtures with geometries as a function of time. This is, by any account, a hugely challenging task. Techniques that are able to image the internal structure of solid objects have had a huge impact on healthcare, the physiological and neurological sciences and more recently materials science [2] , [3] , [4] , [5] , [6] , [7] , [8] , [9] . The more precise and quantitative the information that can be imaged, or spatially mapped, the better. Recently, a number of non-destructive X-ray diffraction (XRD) methods have been developed that allow the mapping of chemical and structural information from bulk objects in three- and four dimensions [10] , [11] . Notably, this includes the development of static and more recently dynamic XRD-computed tomography (XRD-CT) [10] , [11] , [12] , [13] , [14] , [15] , [16] . The latter provides remarkable chemical and physical insight allowing, for example, for the monitoring of evolving solid-state chemistry as well as the mapping of physical quantities such as crystallite size in a spatially resolved way. However, obtaining quantitative structural information for nanoscale objects is a major challenge even without introducing the complexity of performing the measurements under reaction conditions. Because of the disappearance of Bragg peaks for nanosized objects, standard crystallographic methods are no longer suitable, the so-called nanostructure problem; XRD-CT is largely blind to the amorphous and nanocrystalline components of samples [17] . However, emerging methods such as total scattering and the pair distribution function (PDF) methods are producing reliable, quantitative information regarding nanostructure [8] . Many of the heterogeneous devices that we desire to study under in situ or operando conditions, such as batteries, catalytic systems and fuel cells, contain important components that are nanocrystalline. Previous attempts to map amorphous or nanocrystalline components below ~3 nm using XRD-CT were challenging requiring considerable a priori knowledge for the interpretation [13] , [18] . Traditionally, such materials are better studied using spectroscopic methods with, for example, recent techniques such as direct tomography with chemical bond contrast and/or (soft) transmission X-ray microscopy capable of providing the short-range order information necessary to image different amorphous or nanocrystalline components [19] , [20] , [21] . As PDF provides similar information, it can compete with these methods. Furthermore, by virtue of using high-energy X-rays there are advantages in terms of being able to study complex materials in realistic environments. In addition, the technique is not restricted to providing time-resolved chemical insight on only a small proportion of the system (that is, it does not require using a range of energies to tackle multi-element systems) [19] , [20] , [21] , [22] . Total scattering and PDF methods that utilize the entire Bragg and diffuse scattering signal from a sample are emerging as powerful tools for studying nanostructure [8] , [23] . Indeed, such methods have been previously employed in static and more recently in a time-resolved manner to provide insight into systems under reaction conditions [24] , [25] , [26] , [27] . A limitation of these in situ studies is that they yield an average representation of a small part of the sample, and potentially important positional variations in the chemistry across the specimen are lost. Real-world materials are, by accident or design, rarely homogeneous. By combining total scattering techniques with a CT approach, we show how it is indeed possible to obtain and spatially map quantitative structural and nanostructural parameters. As the PDF-CT method yields quantitatively reliable total scattering PDFs in each voxel of the sample, all of the PDF analyses normally carried out, such as model independent analyses of peak positions, heights and widths and nanostructure refinements, may be carried out as a function of position in the sample. Importantly, as rapid acquisition X-ray PDF studies naturally make use of high-energy incident radiation, the method is not limited by the atomic number of the atomic species present and is capable of penetrating relatively thick reactor vessels. The signals from such vessels may swamp the signal from the sample contained within, but with PDF-CT the tomographic reconstruction places these signals into different voxels rendering unnecessary a subtraction of the sample container. The method is therefore optimal for performing studies on systems evolving under process reaction conditions [28] . PDF-CT will undoubtedly have use and application across a wide range of disciplines and represents a significant advance in the field of imaging. Many readers may be familiar with XRD but have not had direct experience with PDF. From an experimental perspective, the latter only requires measurement over a larger momentum transfer ( Q ) range, that is, recording to higher 2 θ . With standard fast in situ XRD, Q will be sampled up to a typical maximum ( Q max ) of perhaps 10 Å −1 . In the equivalent PDF study, this is typically much higher, perhaps 25 or 30 Å −1 . Nevertheless, the PDF measurement data are simply diffraction data (XRD) whereby the PDF is obtained by Fourier transform processing (as is outlined more fully in the Methods section). The PDF simply describes the probability, G , of finding pairs of atoms at a real-space distance r . It does not implicitly contain information about the direction of those vectors with respect to one another, as the data comprise a one-dimensional pattern of the total scattering from all atom pairs present in the material. The results presented herein demonstrate the applicability of the PDF-CT method to obtain ‘local structure’ contrast images from amorphous and nanocrystalline samples that would normally be impossible to image/interrogate by any other method. Demonstration of method with phantom test object To demonstrate the reliability of PDF-CT, a phantom sample composed of a mixture of amorphous and semicrystalline materials was constructed. Silica glass and basalt spheres with polystyrene and poly(methyl methacrylate) fragments were packed together in a 4,4′-oxydiphenylene-pyromellitimide (Kapton) tube. The purpose was to benchmark the PDF-CT method against the established XRD-CT. The images of the distributions of each component are shown in Fig. 1 . The distributions found by XRD-CT are shown ( Fig. 1a–e ) with the Compton scatter shown in ( Fig. 1f ), whereas those found by PDF-CT are shown in ( Fig. 1h–l ) with a false-colour composite image shown in ( Fig. 1m ). They are highly similar indicating that the PDF-CT reconstruction is working well. Representative XRD and PDF patterns from a voxel containing each component are also shown in Fig. 1g,n for comparison, respectively. The PDF-CT images were obtained by fitting a linear combination of the PDFs of each component to the measured PDF in each voxel and then plotting the fraction of each phase as a function of position. The resulting images give a clean separation of the different species present with virtually no misassignment. It is clear from the PDF-CT-derived false-colour composite image ( Fig. 1m ) that all of the constituents have been correctly identified resulting in a space-filled image. Small dark regions between the particles were filled with wax. 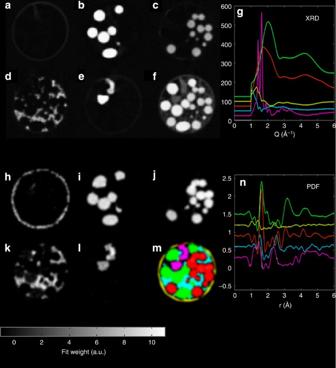Figure 1: Imaging of 2.75 mm diameter test object. Distributions of Kapton, basalt, silica glass, polystyrene and PMMA as determined by XRD-CT (a–e, respectively) and the PDF-CT (h–l, respectively); all images are presented with a common linear grey-coloured scale bar. The image (f) is obtained from the very highQdiffraction signal, which is dominated by Compton scattering, and therefore represents the sample electron density image. The image (m) is the colour-coded composite image derived from components (h–l) determined by PDF-CT; it is coloured accordingly: yellow (Kapton), green (basalt), red (glass), pink (polystyrene) and PMMA (cyan). The line graphs ingandnshow portions of XRD and PDFs, respectively, for the individual components coloured in accordance with the composite image (m). CT, computed tomography; PDF, pair distribution function; PMMA, (poly(methyl methacrylate)); XRD, X-ray diffraction. Figure 1: Imaging of 2.75 mm diameter test object. Distributions of Kapton, basalt, silica glass, polystyrene and PMMA as determined by XRD-CT ( a – e , respectively) and the PDF-CT ( h – l , respectively); all images are presented with a common linear grey-coloured scale bar. The image ( f ) is obtained from the very high Q diffraction signal, which is dominated by Compton scattering, and therefore represents the sample electron density image. The image ( m ) is the colour-coded composite image derived from components ( h – l ) determined by PDF-CT; it is coloured accordingly: yellow (Kapton), green (basalt), red (glass), pink (polystyrene) and PMMA (cyan). The line graphs in g and n show portions of XRD and PDFs, respectively, for the individual components coloured in accordance with the composite image ( m ). CT, computed tomography; PDF, pair distribution function; PMMA, (poly(methyl methacrylate)); XRD, X-ray diffraction. Full size image If the intention is simply to image the location of different components, this example illustrates that even when they are amorphous or semicrystalline, images can be obtained by XRD-CT when the constituents are known. On the other hand, PDF data provide detailed structural information enabling component finger printing as well as supplementary chemical information, for example, information about coordination and oxidation state. In many cases, the nature of the shortest chemical bond is sufficient to distinguish between glass ( Q ~1.61 Å because of tetrahedral Si–O species), poly(methyl methacrylate) ( Q ~1.52 Å because of tetrahedral sp 3 C–C species) and Kapton ( Q ~1.40 Å reflecting an ‘average’ nearest neighbour distance dominated by the 18 sp hybridized C–C species). Distinguishing between species that possess similar scattering pairs (that is, between glass and basalt with Si–O contributions at Q ~1.61 Å) requires a further inspection of the PDF to higher r , which reveals that the more crystalline basalt possesses a stronger contribution at 3.10 Å (Si–Si) [29] , [30] . This experiment serves to illustrate clearly that phases can indeed be mapped, separated and then identified by the PDF-CT method, opening up the possibility of chemical bond or chemical species contrast tomography applicable irrespective of kinetic state. In situ study of Pd/Al 2 O 3 industrial catalyst body We now turn our attention to a scientifically and technologically important example: the formation of nanocrystalline material within an industrial Pd-containing γ-Al 2 O 3 catalyst body. Catalyst bodies are mm-sized porous support units (typically cylinders/spheres) onto which metals and metal oxides are deposited for the purpose of performing large-scale industrial catalysis. They are loaded in their thousands into industrial catalytic reactor units as catalyst beds. The functioning of the bed and hence the efficiency of the entire industrial process is dependent on the performance of the catalytic body per se and as such it becomes extremely pertinent to understand how they are prepared and operate in practice. It is estimated that upwards of 85% of the chemicals we utilize on a daily basis will have come into contact with an industrial heterogeneous catalyst of some type in one form or another at some point in their manufacture; hence, their significance both in environmental and economic terms should not be underestimated [31] . The catalyst body serves some basic functions: it provides a fairly inert (and as such robust to the rigors of the industrial process) gas porous microstructure onto which a catalyst can be thinly dispersed and fixed in position by chemical bonding to the substrate. By choice of preparation route, the catalyst can be directed to a desired distribution to maximize efficiency, both in terms of producing the desired industrial product and also minimizing the amount of catalyst used [32] , [33] , [34] , [35] . For example, Pd (an expensive material) catalysts are employed for both hydrogenation and oxidation reactions [36] , [37] , [38] , [39] . To date, X-ray methods have been used to image catalyst bodies under both preparation and operation conditions [16] , [40] , [41] , [42] , [43] . The diffraction-based methods, the most insightful to date, are however limited to the bulk state. However, by their very nature, catalytic materials are most often most efficacious when deposited in a nanocrystalline form and then often with particle sizes<10 nm [44] , [45] . Even then, the very active species are smaller still, often beyond the range observable with XRD, thus rendering the most interesting and important species unobservable by conventional imaging [46] . PDF-CT offers a new opportunity to examine these important materials. Catalyst bodies were loaded with palladium and XRD patterns were measured at beamline ID15A of the European Synchrotron Radiation Facility using an XRD-CT tomographic data collection protocol, as described in Methods. The XRD recorded from this sample were reconstructed. The reconstructed XRD is a subset of the PDF measurement utilizing the low Q region of the data, where Q is the magnitude of the scattering vector ( Q =4 π sin θ / λ ). It can be used to look at the distribution of crystalline components within the sample. Supplementary Fig. S1 shows a comparison of micro-CT (μ-CT) and XRD derived from the PDF-CT image data. As to be expected, there is good correlation between the images derived by both methods. The μ-CT reveals that a significant portion of material is deposited at the periphery of the sample (termed an eggshell distribution); see Supplementary Fig. S2 for an explanation of catalyst distribution types. An important benefit of the CT approach is that it is possible to distinguish scatter derived from the sample and that derived from sample holders/reaction chambers; this is demonstrated in Supplementary Fig. S3 where we see that the glass cell is clearly spatially distinguished from the sample. 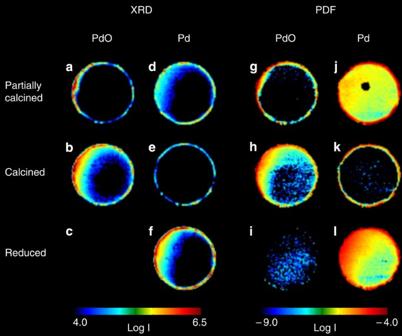Figure 2: Comparison of XRD-CT and PDF-CT. Comparison of information from XRD-CT and PDF-CT during calcination and reduction of 3 mm Ø Pd/Al2O3industrial catalyst. The XRD-CT intensity maps are determined from the profiled intensities of the (002) and (111) reflections of PdO (a–c) and fcc Pd (d–f), respectively. The PDF-CT intensity maps are determined from the profiled intensities of the Pd–Pd scattering pairs at 3.44 and 2.71 Å as representative of PdO (g–i) and fcc Pd (j–l), respectively. The black circle visible injof the partially calcined sample corresponds to a void in the sample. This is not visible in the calcined and reduced samples as measurements were performed at a different height on the sample; this is explained inSupplementary Fig. S1. PDF-CT identifies both Pd and PdO material unseen in the XRD-CT but visible in the μ-CT. Images derived from XRD and PDF are each presented with a common log colour-scale; scale bars for each set are shown at the bottom of the figure. CT, computed tomography; fcc, face centred cubic; PDF, pair distribution function; XRD, X-ray diffraction. Figure 2a–f shows the reconstructed distributions of crystalline phases present derived from the ‘diagnostic’ (002 and 111) reflections of PdO ( Fig. 2a–c ) and face centred cubic (fcc) Pd ( Fig. 2d–f ), respectively. Figure 2g–l shows the reconstructed distributions of selected atomic scattering pairs pertaining to the same crystalline phases, for example, the components with peaks at 3.44 and 2.71 Å in the radial distribution functions due to Pd–Pd pairs in PdO ( Fig. 2g–i ) and fcc Pd ( Fig. 2j–k ), respectively. Representative diffraction patterns and PDFs from different portions of the sample in the various states can be found in Supplementary Figs S4 and S5 . It should be noted that there is a strong signal from the γ-Al 2 O 3 support in every voxel, which must be subtracted before the patterns from the Pd/PdO contributions can be clearly observed. Despite these challenges, which are common in this kind of study, the results are successful. In the partially calcined state, the XRD-CT map in Fig. 2a,d confirms that the cause of the eggshell distribution seen in the μ-CT is the presence of large amounts of both PdO and Pd phases at the sample periphery. Importantly, although this eggshell distribution is also observed in the PDF-CT data, the technique also reveals a number of ‘diffraction silent’ metallic Pd particles beyond the sample periphery and inside the catalyst body. The observation of metallic Pd on the inside most probably occurs as a result of thermal decomposition of the complex in the comparatively (relative to the periphery) oxygen-poor environment. This interpretation is supported by the observation of a halo of unreduced metallic Pd penetrating into the interior of the catalysis body in the XRD-CT image in the partially reduced state, which disappears on further calcination. Figure 2: Comparison of XRD-CT and PDF-CT. Comparison of information from XRD-CT and PDF-CT during calcination and reduction of 3 mm Ø Pd/Al 2 O 3 industrial catalyst. The XRD-CT intensity maps are determined from the profiled intensities of the (002) and (111) reflections of PdO ( a – c ) and fcc Pd ( d – f ), respectively. The PDF-CT intensity maps are determined from the profiled intensities of the Pd–Pd scattering pairs at 3.44 and 2.71 Å as representative of PdO ( g – i ) and fcc Pd ( j – l ), respectively. The black circle visible in j of the partially calcined sample corresponds to a void in the sample. This is not visible in the calcined and reduced samples as measurements were performed at a different height on the sample; this is explained in Supplementary Fig. S1 . PDF-CT identifies both Pd and PdO material unseen in the XRD-CT but visible in the μ-CT. Images derived from XRD and PDF are each presented with a common log colour-scale; scale bars for each set are shown at the bottom of the figure. CT, computed tomography; fcc, face centred cubic; PDF, pair distribution function; XRD, X-ray diffraction. Full size image After further calcination, as expected, metallic Pd is oxidized to PdO. However, it is clear from both XRD- and PDF-CT that metallic Pd persists in the eggshell with a slightly higher loading of Pd/PdO towards the top left hand side. The particle size in the eggshell region is large, as the signal is clearly seen in XRD-CT and presumably originates from the large Pd particles that are not fully oxidized. However, strikingly, the metallic Pd in the core of the catalyst body coming from diffraction-silent small particles is now removed by this calcining process and replaced with PdO. Finally, in the reduced state (after treatment in H 2 ) the PdO is seen to diminish completely yielding crystalline fcc Pd, with this phase again being located predominantly at the periphery and then preferentially on the left. Although PDF-CT data are consistent with this observation, a smattering of unaccounted for signal intensity within the main body of the sample because of both Pd and PdO suggests that the conclusions drawn from XRD-CT are not entirely complete; ‘diffraction-silent’ (nano)material is again present. The previous observation that the diffraction-silent PDF-CT signal in the core of the catalyst is from small nanoparticles is verified by further quantitative analysis. In nanomaterials, peaks in the PDF diminish in intensity as a function of r because of finite size effects. This happens with a characteristic functional form depending on the particle shape and size, and can be used to determine the crystallite size. Representative PDFs from voxels in the eggshell and in the core are shown in Fig. 3b,c , respectively. By direct inspection, it is apparent that the PDF signal is dying out more quickly in the latter case, and as a consequence the diffraction-silent nanoparticles in the centre of the catalyst body must be very small. It is possible to model this by applying the characteristic function for a sphere to the calculated PDF, resulting in a good fit for a visible nanoparticle diameter of ~1.4 nm in this particular case. On the other hand, the particles located in the shell exceed ~4 nm. Importantly, this analysis process can be applied to all the voxels to extract a map of particle size. 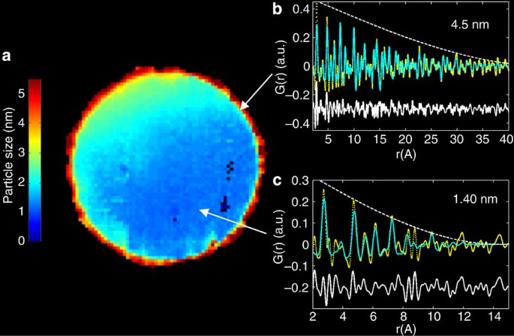Figure 3: Pd particle size distribution. (a) Distribution of particle sizes of fcc Pd within the catalyst body under reducing conditions. Portions of the PDF data for selected pixels at the edge (b) and interior (c) of the catalyst body (yellow data points) with an fcc model fit (cyan) and difference (white). The dashed white line indicates the radial-dependent crystallite size damping factor. fcc, face centred cubic; PDF, pair distribution function. Figure 3: Pd particle size distribution. ( a ) Distribution of particle sizes of fcc Pd within the catalyst body under reducing conditions. Portions of the PDF data for selected pixels at the edge ( b ) and interior ( c ) of the catalyst body (yellow data points) with an fcc model fit (cyan) and difference (white). The dashed white line indicates the radial-dependent crystallite size damping factor. fcc, face centred cubic; PDF, pair distribution function. Full size image This study has demonstrated the feasibility and power of PDF-CT for the identification and characterization of materials that lack long-range order within the interiors of bulk objects. The catalyst body study clearly demonstrates that the picture obtained by traditional μ-CT and XRD-CT is limited to cases where the amount of material present is sufficient and the crystalline component is of sufficient size or order. The PDF-CT method by contrast provides a much more complete depiction providing information on both the chemical and physical state of the phases present regardless of particle size. In this study, we demonstrate that very small nanocrystalline Pd and PdO materials are present in the interior of the sample. The particle size in the eggshell at the surface is ~4 nm but the average particle diameter falls quickly to ~1.4 nm within a distance of a few tens of microns from the surface and even smaller on moving to the interior of the catalysis body. Importantly, when trying to correlate structure with function in materials science during process operation such as in catalytic applications, the presence of a distribution of species is almost unavoidable but it is difficult to detect and characterize. However, this information is vital when trying to determine the nature of the active species, particularly so when it has been shown that very small crystallite sizes can be extremely active [46] , [47] , [48] , [49] . In the present study, it is not clear whether the significant catalytic activity would originate from the larger and more numerous particles located in the eggshell at the periphery of the body or by the smaller ones in the interior. However, by using dynamic PDF-CT, it is now possible to provide a more complete picture of the catalyst sample and the evolutionary processes by which it develops in terms of the species that form and their physical properties, rendering this the preferred technique to allow us to develop more robust structure–activity relationships in the future in real catalyst samples and ultimately to guide catalyst design. PDF-CT is not limited to the study of catalysts and we expect the method to have application to many other fields of research, for example, biomaterials, materials science, chemistry, geology, environmental science, palaeontology and cultural heritage. The relatively fast acquisition times associated with collection mean that high-resolution imaging in two-dimensional and three-dimensional (4D), or else time-resolved imaging, is currently possible, as has been demonstrated with conventional XRD-CT [15] . No one technique can provide all of the information required to fully characterize an unknown sample. PDF-CT in the form presented herein, however, can be considered a dual technique: the reconstructed XRD-CT being a subset of the PDF-CT enables direct extraction of any Bragg signal that may be present. Indeed, an experiment can be optimized to maximize the data quality and recorded q -spacing range to reflect the types of material under study. Being a tomographic technique, the number of components within a selected volume element is most likely greatly reduced from the number present within the whole sample (certainly, for example, being free from contributions from sample containers/environmental cells). Thus, the individual reconstructed XRD and PDF are likely simplified and information within them more readily extracted. This can make identification easier when there is limited a priori information. One can also consider extending the method further by combining existing imaging techniques, for example, tomographic X-ray absorption spectroscopy [43] ; this could also be realized by performing anomalous or diffraction anomalous fine structure-type PDF-CT to yield the additional voxel-specific spectroscopic information. PDF-CT will have big advantages over existing methods in a range of applications: it utilizes high-energy X-rays and as such can be used to probe inside opaque and dense apparatus; it does not have to be conducted around an elemental X-ray absorption edge; it makes use of standard recording equipment, not requiring a specially designed diffractometer or high-resolution lenses. With modern synchrotron sources, submicron beams are becoming more widely available allowing for the possibility of PDF-CT imaging with resolution on the nanometre scale in the near future [50] . With the projected developments in source and detector technology, it may replace μ-CT and XRD-CT as it can measure both crystalline and nanocrystalline components, and their mixtures, to become the preferred X-ray imaging tool offering unprecedented insight into the structure and properties of materials across the medical and materials science spectrum [51] , [52] . PDF-CT provides a real-space technique capable of generating bond-length contrast images, and has the potential to replace the conventional X-ray image measurement. Data collection The PDF tomography-computed experiments were performed at the ID15A beamline of the European Synchrotron Radiation Facility. X-rays were produced using an undulator insertion device with a gap of 6.25 mm and focused using a set of aluminium and beryllium refractive X-ray lenses (a so-called transfocator). Monochromatic E =69.95 KeV X-rays were selected using a bent (to increase X-ray flux) Laue Geometry double crystal monochromator yielding a bandwidth of ca. 300 eV. The focused spot size at the sample position was 30 μm vertical and 120 μm horizontal. The horizontal beam size was then further reduced using a set of horizontal slits, and the final beam size was 30 × 50 μm 2 . A Debye–Scherrer (transmission) geometry was employed with diffracted X-rays recorded on a Trixell Pixium 4700 flat panel digital detector. Supplementary Fig. S6 shows photographs of the experimental set-up indicating positions of various components. A thick walled brass tube terminating in a 1-mm pinhole was placed just before the sample to reduce air scattering. Samples were mounted and aligned via a goniometer. For the in situ experiments, samples were mounted in a quartz glass tube. Heating was achieved with two Le Mini programmable air heat guns, and gas was delivered to the sample via a gas stub; the temperature inside the quartz tube was calibrated using a thermocouple. The goniometer was mounted to a rotation stage, which in turn was mounted to a linear stage (with travel perpendicular to the beam in the horizontal plane). A small tungsten beam stop of diameter 2 mm was placed a few centimetres behind the sample. The sample-detector distance was adjusted such that the maximum measured Q ( Q max ) was ~30 Å −1 . Calibration of this distance, and the orthogonality of the detector to the incident beam, was performed using a NIST CeO 2 diffraction standard. In all PDF tomography experiments, a tomographic data set was obtained by completing a series of line scans covering an angular range from 0° to 180°. For all scans, a collection strategy was employed to obtain a 50-μm 2 pixel size in the reconstructed image. We typically collected ~80 diffraction patterns in an approximately 4 mm line scan with 60 different projections, corresponding to an angular step of 3°. Data processing Each two-dimensional diffraction pattern was pre-processed to correct for detector flat field variations, geometry and beam polarization, and was then azimuthally integrated to produce a projection set consisting of one-dimensional diffraction patterns of intensity versus scattering vector amplitude. A tomographic reconstruction algorithm (filtered back projection) was then applied for each point of the scattering pattern to obtain the diffraction pattern in each specific volume element of the sample. This resulted in ~10 4 distinct diffraction patterns, which were processed to obtain the PDF using the recently developed rapid and automatable PDFgetX3 program based on a novel algorithm [53] . The PDF, G ( r ), is obtained from the sine-Fourier transform of the total scattering structure function, S ( Q ), which is the properly corrected and normalized powder diffraction intensity according to refs 54 , 55 , 56 . In practice, the integral in equation (1) is limited to a maximum Q = Q max . G ( r ) represents the probability of finding an atom at a given distance ‘ r ’ from another atom. The relative intensity in the PDF relates directly to the number of these pairs and their scattering power. For nanostructured materials, the intensities of the PDF peaks diminish with increasing r because of the finite size of the objects (or more strictly the finite range of the structural coherence). The point at which peaks disappear in the PDF indicates the diameter of the largest extent of the structural order in the material and this can be used to ascertain whether a material is amorphous or nanocrystalline (or indeed highly crystalline). For a crystalline material, in principle, the PDF peaks persist indefinitely, but in practice fall off because of the finite resolution of the diffraction measurement. Once resolution effects are corrected by measuring the PDF of calibration materials, accurate crystallite sizes may be deduced by fitting the data. The PDF data sets were modelled using structure refinement methods implemented in the PDFgui package [53] . Study of Pd industrial catalyst body A batch of five Pd catalyst bodies were prepared by pore-volume impregnation with Pd(NH 3 ) 4 Cl 2 .H 2 O pre-cursor (110 μl of a 4 wt% solution). These were shaken for 5 min, dried (120 °C for 120 min) and then calcined (ramp 50–500 °C at 4.5 °C min −1 ; hold 60 min at 500 °C; cool down at 4.5 °C min −1 ). A single catalyst body was selected from this batch and mounted within the in situ set-up, and then scanned using the PDF tomography method. Next, the selected catalyst body was subjected to a long calcination (ramp 20–500 °C at 4.5 °C min −1 ; hold 180 min at 500 °C; cool down at 25 °C min −1 ) in situ after which the sample was again scanned. Finally, the sample was put under 5% H 2 /Ag and again scanned. Post experiment, the catalyst body was examined non-destructively by conventional μ-CT. How to cite this article: Jacques, S. D. M. et al . Pair distribution function-computed tomography. Nat. Commun. 4:2536 doi: 10.1038/ncomms3536 (2013).